GaAs nanopillar-array solar cells employingin situsurface passivation Arrays of III–V direct-bandgap semiconductor nanopillars represent promising photovoltaic candidates due to their inherent high optical absorption coefficients and minimized reflection arising from light trapping, efficient charge collection in the radial direction and the ability to synthesize them on low-cost platforms. However, the increased surface area results in surface states that hamper the power conversion efficiency. Here, we report the first demonstration of GaAs nanopillar-array photovoltaics employing epitaxial passivation with air mass 1.5 global power conversion efficiencies of 6.63%. High-bandgap epitaxial InGaP shells are grown in situ and cap the radial p–n junctions to alleviate surface-state effects. Under light, the photovoltaic devices exhibit open-circuit voltages of 0.44 V, short-circuit current densities of 24.3 mA cm −2 and fill factors of 62% with high external quantum efficiencies >70% across the spectral regime of interest. A novel titanium/indium tin oxide annealed alloy is exploited as transparent ohmic anode. Nanometer-scaled materials [1] , [2] , [3] , [4] , [5] , [6] , [7] , [8] , [9] , [10] , [11] , [12] , [13] , [14] , [15] are attractive candidates to implement efficient designs for the conversion of solar energy to electricity. Colloidal quantum dots [16] , [17] , nanoparticles [18] , [19] , nanodomes [20] and nanowires [1] , [2] , [3] , [4] , [5] , [6] , [7] , [8] , [9] , [10] , [11] , [12] , [21] , [22] , [23] are actively investigated to improve the charge collection process along with broadband-enhanced light absorption [24] resulting from their optical trapping properties. The adoption of such materials is ultimately aimed to reduce the cost while improving the total power conversion efficiency (PCE) of the final device. In core–shell p–n junctions embedded within nanopillars (NPs), the electron-hole pair separation occurs in the radial direction and the photogenerated carriers have to travel distances much shorter than the minority carrier diffusion length [23] , [25] . Considering that the photo-active region is represented by the nanostructures themselves, the NP arrays can be embedded in a flexible and transparent polymer (for example, polydimethylsiloxane) and peeled off from the growth substrate, which can be re-used in subsequent growth runs [26] , lowering fixed costs in manufacturing productions. III–V direct-bandgap compound semiconductors offer the chance to efficiently absorb most of the incoming photons within a couple of microns of material thickness and they enable multi-junction integration for a complete ultraviolet/visible/infrared spectral utilization. The high surface-to-volume ratio represented by the adoption of a cylindrical radial junction increases both the active depletion region as well as the overall surface area of the device, which then becomes more susceptible to recombination of photogenerated charge carriers. Because of the surface-state charges arising from surface scattering, charge recombination and Fermi level pinning, the charge-carrying volume in the NP is much narrower compared with its physical volume, confining the carriers to a smaller conducting core [27] . The high surface recombination velocity results in the annihilation of minority carriers, which would otherwise contribute to a portion of the output in the photovoltaic (PV) device. Recent reports on ensemble of core–shell GaAs nanowires applied to solar cells have revealed conversion efficiencies ranging from 0.83% (ref. 5 ) for as-grown devices to 2.54% (ref. 6 ) for devices post-treated with ammonium sulphide agents. In situ passivating techniques are widely adopted in planar optoelectronic designs to most effectively reduce the surface state density, offering the highest stability over time. Generally, thin layers of epitaxial high-bandgap materials act as a barrier to prevent carriers from recombining at the surface [28] , [29] , [30] . In situ NP passivation represents a challenging task due to the different crystallographic directions [31] , [32] and energetics on the NP facets, while maintaining a lattice-matched growth between dissimilar materials. Hence, there has been no demonstration of integrating in situ epitaxial passivation into radial-junction NP arrays for PV application thus far. Optically, vertically aligned semiconducting wires can trap solar irradiation [11] , [12] more effectively with respect to planar PV designs, and periodic patterns of dielectric spheres and metal particles [13] have shown to increase the probability of photon absorption. Theoretical calculations of periodic arrays of silicon wires [33] reveal a light absorption strongly tunable with respect to the geometric properties of the nanostructures (for example, orientation, diameter, height, filling ratio). Therefore, the adoption of a growth mask on which the various geometric parameters can be determined a priori represents a solution for a controlled NP positioning. In this work, we experimentally demonstrate in situ epitaxial surface passivation of direct-bandgap GaAs NP solar cells via patterned, catalyst-free, selective-area epitaxy (SAE) [6] , [34] . High-bandgap InGaP shells are grown in situ and lattice-matched on the GaAs NPs to prevent from high surface recombination rates and Fermi level pinning [30] . The patterned growth mask is optimized in terms of NP pitch and tiling pattern to maximize the enhanced optical absorption of the arrays. All devices employ a novel titanium (Ti)/ indium tin oxide (ITO) annealed alloy as transparent ohmic anode. Maximizing the optical absorption using numerical simulations Before growth, full-wave finite-difference time-domain simulations (software Lumerical) are implemented to investigate/optimize the enhanced absorption with respect to the geometrical parameters available in the growth mask design, to achieve near-perfect absorption while minimizing material usage. Tiling pattern and centre-to-centre pitch are considered as variables in this set of simulations and the optimized topology can be fabricated by means of the SAE growth approach. A limited number of reports of optical absorption modelling are presented in literature for periodic arrays of III–V NPs. Geometrical tuning of InAs nanowires [3] is demonstrated both experimentally and theoretically for square-tiling patterns. Periodic arrays of GaAs NPs are investigated in terms of optical absorption with varying diameter-over-pitch ratios [4] , in square pattern arrangements. The reports pervasively consider bare periodic arrays of nanowires (not sufficient for a practical nanowire solar cell). Hence, it is necessary to model the optical properties of the final device. 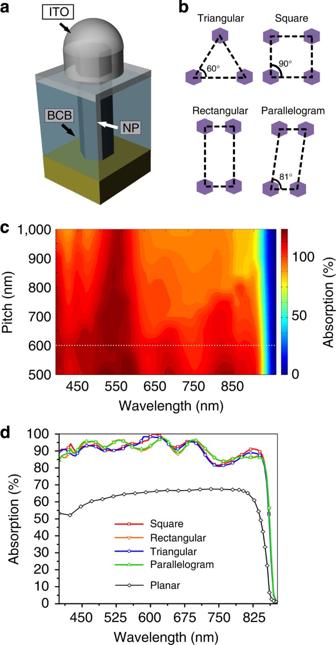Figure 1: Tailoring the optical absorption using numerical simulations. (a) Three-dimensional schematic of the complete structure used in the finite-difference time-domain simulations. To notice, the NP is embedded in the BCB layer and capped by a conformal layer of ITO as transparent top electrode. (b) Unit cells of triangular, square, rectangular and parallelogram tiling patterns are investigated. (c) 2D contour plot of NP pitch P (500 nm≤P≤1,000 nm) and wavelength-dependent optical absorption. Red colour indicates high absorption and blue colour corresponds to low absorption. (d) Wavelength-dependent absorption as a function of different tiling patterns for a fixed 600-nm pitch (dashed cutline fromFig.1c). Figure 1a represents the three-dimensional (3D) schematic of the complete, fully processed simulated structure. Figure 1b displays the triangular, square, rectangular and parallelogram lattice geometries. The incident light contains both x and y polarizations to better match the unpolarized solar spectrum. Periodic boundary conditions are considering an infinite array of NPs. The NP height and diameter are fixed at 1.3 μm and 260 nm, respectively. Figure 1c represents a 2D contour plot of wavelength-dependent absorption (400 nm–900 nm) as a function of centre-to-centre pitch (500 nm–1,000 nm) with a colour legend spanning from low absorption (dark blue) to high absorption (dark red) values. The plot shows that, with lower pitch size or equivalently a higher filling ratio, the absorption of the periodic structure increases. The result is expected owing to the fact that optical resonance-guided modes increase the electromagnetic light intensity, resulting from the coupling of the normally incident light to high-Q leaky modes of the periodic structure [35] . For decreasing pitch values, the light is greatly confined in the NP array and excites optical resonance-guided modes [36] , [37] , which in turn greatly enhance the optical absorption. Hence, a pitch size of 600 nm is chosen here as an optimized device dimension, also considering that radii below 100 nm can hardly accommodate quasi-neutral regions on both core and shell sides for an efficient carrier extraction at the ohmic electrodes. In Fig. 1d , four different tiling patterns (as shown in Fig. 1b ) with optimized 600 nm pitch are compared with respect to GaAs planar substrates. The areas for the unit cell in all four patterns are identical (600 nm × 600 nm); as a result, the filling ratio is kept constant, and only the effect of tiling pattern is taken into account in this comparison. From the simulations, it can be concluded that tiling pattern does not substantially change the absorption spectrum compared with pitch size, or filling ratio, which is the governing factor in determining the absorption efficiency. Slight variations are attributed to the differences in the symmetry of the geometries. This result is non-trivial in light of the fact that previous works [38] on periodic non-subwavelength silicon microwires (several microns for both pitch and diameter) exhibited varying optical properties depending on the periodic arrangement adopted. Figure 1: Tailoring the optical absorption using numerical simulations. ( a ) Three-dimensional schematic of the complete structure used in the finite-difference time-domain simulations. To notice, the NP is embedded in the BCB layer and capped by a conformal layer of ITO as transparent top electrode. ( b ) Unit cells of triangular, square, rectangular and parallelogram tiling patterns are investigated. ( c ) 2D contour plot of NP pitch P (500 nm≤ P ≤1,000 nm) and wavelength-dependent optical absorption. Red colour indicates high absorption and blue colour corresponds to low absorption. ( d ) Wavelength-dependent absorption as a function of different tiling patterns for a fixed 600-nm pitch (dashed cutline from Fig.1c ). Full size image NP-array growth and device fabrication The growth structure for GaAs NP solar cells is presented in Fig. 2a . The III–V NPs are formed by catalyst-free, selective-area metal organic chemical vapour deposition on masked n + -doped (111)B GaAs substrates. Tetra-ethyl-tin and di-methyl-zinc are chosen as n-type and p-type dopants and calibrated flow rates from planar test measurements are selected to achieve carrier densities of N a,core =1 × 10 17 cm −3 and N d,shell =1 × 10 18 cm −3 , respectively ( Supplementary Fig. S1 and Supplementary Discussion). Once the radial p–n junction is formed, an InGaP shell lattice matched to GaAs is grown. In this fashion, an estimated GaAs core diameter of 180 nm, GaAs shell thickness of 40 nm ( Supplementary Fig. S2 and Supplementary Discussion) and InGaP-passivating shell of 5 nm are formed, with a final NP height of 1.3 μm (see Methods). The growth conditions are reported in more details elsewhere [34] . The InGaP layer results into a negligible absorption for such thin epitaxial window. The total active area amounts to 500 μm × 500 μm and is univocally defined during the patterning process. 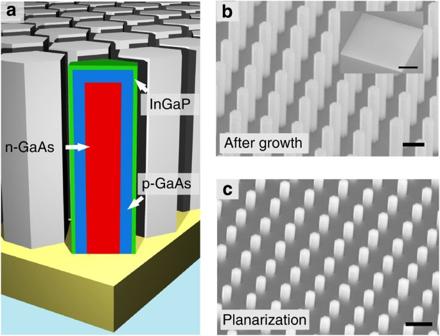Figure 2: SAE NP array. (a) Schematic drawing of the GaAs radial p–n junctions with the InGaP-passivating shell (not to scale). (b) A 45°-tilt scanning electron microscope image of a typical array of GaAs NPs grown by metal organic chemical vapour deposition technique with an optimized 600 nm pitch. Scale bar, 400 nm. Inset: selective-area epitaxial approach allows to position the array and define the growth arrangement by means of a patterned dielectric mask onto the substrate. Scale bar, 150 μm. (c) A 45°-tilt scanning electron microscope image of an NP array after planarization and subsequent etch-back. This step is necessary to spatially separate the anode from the cathode in the photovoltaic cells to prevent top–bottom shunting. Scale bar, 600 nm. Figure 2b shows a 45°-tilted scanning electron microscope image of typical in situ passivated GaAs core–shell NP arrays after epitaxy. The growth is uniform across the whole masked area as it appears from the inset. Subsequent to SAE, ohmic bottom contacts are formed by annealing a gold-germanium/nickel/gold metal alloy to the highly doped substrates. The NP arrays are then planarized with benzocyclobutene (BCB) that represents a transparent electrical insulator to well separate in space the top anode from the bottom cathode. After hard curing and dry etch-back of the BCB, ~350 nm of the NP tips are exposed and ready to be contacted as displayed in Fig. 2c . BCB represents a suitable planarizing polymer with optical transparency in excess of 99% ( http://www.dow.com/cyclotene/solution/optical.htm ). Figure 2: SAE NP array. ( a ) Schematic drawing of the GaAs radial p–n junctions with the InGaP-passivating shell (not to scale). ( b ) A 45°-tilt scanning electron microscope image of a typical array of GaAs NPs grown by metal organic chemical vapour deposition technique with an optimized 600 nm pitch. Scale bar, 400 nm. Inset: selective-area epitaxial approach allows to position the array and define the growth arrangement by means of a patterned dielectric mask onto the substrate. Scale bar, 150 μm. ( c ) A 45°-tilt scanning electron microscope image of an NP array after planarization and subsequent etch-back. This step is necessary to spatially separate the anode from the cathode in the photovoltaic cells to prevent top–bottom shunting. Scale bar, 600 nm. Full size image Transparent ohmic contact as an efficient hole collector The ITO/GaAs interface has been reported in several works to be either ohmic [39] or Schottky [40] , [41] depending on deposition conditions and post-deposition treatments. Although characterized by n-polarity, ITO films can result into either Schottky or ohmic contacts to both n- and p-GaAs. To achieve an ohmic interface, high annealing temperatures are necessary (550–700 °C). This could detriment the epitaxial NP crystal grown at comparable temperatures. Conversely, rectifying contacts resulting from parasitic Schottky barriers can create wide depletion regions, forcing the carriers to overcome the potential barrier by thermionic emission [42] . Despite fundamental, these transport properties at the electrode interface have been so far overlooked, and only a few theoretical reports discuss these effects in GaAs nanowire-based solar cells [43] . With metals, Ti/gold ohmic contacts to p-GaAs are routinely achieved with very low resistance [44] , without requiring any thermal annealing step. For this reason, Ti(4 nm)/ITO(350 nm) thin films are RF sputtered and calibrated on p-GaAs substrates ( N sub ~10 18 cm −3 ) at room temperature in one single run to prevent oxidation of the Ti layer. Plasma-assisted sputtering is chosen here as it forms a 3D wrap-around contact to ensure a uniform carrier extraction. The deposition is divided into two major segments. First, a continuous metallic Ti thin film is deposited at low deposition rates (~1 nm/min). Second, a 350-nm ITO overlayer is sputtered (see Methods). Subsequently, current–voltage ( I–V ) measurements are carried out to assess the transport properties of the multi-layered electrode. 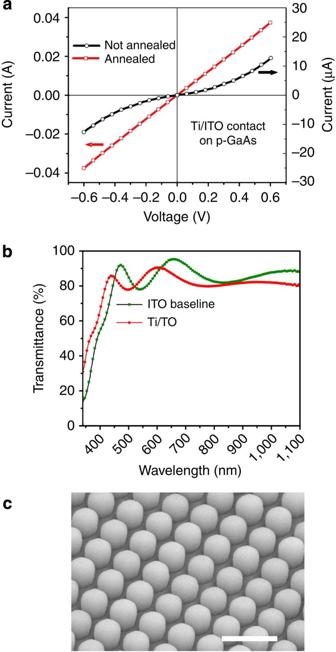Figure 3: Optoelectronic characterization of transparent electrode. (a) Current–voltage measurements of sputtered Ti/ITO alloy on p-type GaAs exhibiting a clear back-to-back Schottky characteristic before thermal annealing (black circles). Subsequent to a 300 °C treatment, an ohmic behaviour is observed with high conduction currents across the transparent contact/semiconductor interface (red squares). (b) Fourier transform infrared spectroscopy measurements of optical transmittance for a standard indium tin oxide baseline compared with a Ti/ITO film (both on quartz slides). A thin titanium interlayer (~4 nm) still ensures an acceptable optical transparency over the spectral regime of interest. (c) Scanning electron microscope image of sputtering deposition which exhibits a uniform, wrap-around contact morphology at the NP tips. Scale bar, 600 nm. Figure 3a plots out the I–V characteristics. The as-sputtered Ti/ITO film exhibits a clear Schottky behaviour, with conduction currents in the microampere range. After low-temperature (300 °C) thermal annealing, the contact shows remarkable ohmic properties, with current values in fractions of ampere range. Figure 3b shows Fourier transform infrared spectroscopy measurements (from 340 nm–1100, nm wavelength) of optical transmittance for a standard ITO baseline compared with a Ti/ITO film (both on quartz slides). Despite a small transmittance drop, the optimized electrode is highly transparent and therefore can be utilized to contact the p-GaAs shells in the NP arrays. Following a selective chemical wet etch of the InGaP shells at the NP tips ( Fig. 2c ), the Ti/ITO alloy is conformally deposited as top anode as shown in the inset of Fig. 3b and thermally annealed with a four-probe-measured sheet resistance of 12.5 Ω/□. Figure 3: Optoelectronic characterization of transparent electrode. ( a ) Current–voltage measurements of sputtered Ti/ITO alloy on p-type GaAs exhibiting a clear back-to-back Schottky characteristic before thermal annealing (black circles). Subsequent to a 300 °C treatment, an ohmic behaviour is observed with high conduction currents across the transparent contact/semiconductor interface (red squares). ( b ) Fourier transform infrared spectroscopy measurements of optical transmittance for a standard indium tin oxide baseline compared with a Ti/ITO film (both on quartz slides). A thin titanium interlayer (~4 nm) still ensures an acceptable optical transparency over the spectral regime of interest. ( c ) Scanning electron microscope image of sputtering deposition which exhibits a uniform, wrap-around contact morphology at the NP tips. Scale bar, 600 nm. 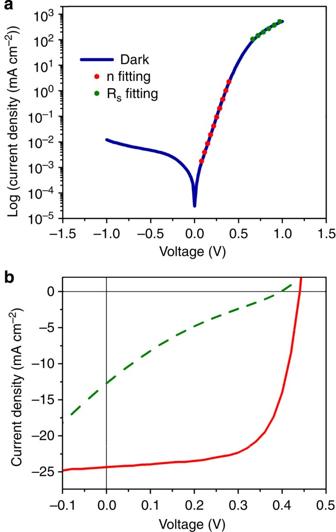Figure 4: Dark and light characterization of photovoltaic devices. (a) Semi-log dark current–voltage characteristic of a typical GaAs NP array. Both ideality factors (n=1.58, red dots) and high-injection series resistance (Rs~530 Ω, green dots) are extrapolated by means of fitting curves. The type of carrier transport is well below the space-charge-limited model (n2). The good diodic behaviour is corroborated by a 104.7rectification ratio. (b) Current density–voltage characteristics under air mass 1.5 global illumination conditions for photovoltaic devices with (solid red line) and withoutin situInGaP shell (dashed green line). InGaP-passivated photovoltaic cells show an open-circuit voltage of 0.44 V, short-circuit current density of 24.3 mA cm−2and FFs of 62%. This translates into a PCE that amounts to 6.63%. Full size image Enhanced PCE using InGaP passivation Figure 4a displays the current density–voltage characteristic under dark of a typical, fully processed, GaAs core–shell NP solar cell with InGaP-passivating shell. The data is plotted in semi-log axis to correctly extrapolate reverse bias leakage current, rectification ratio, ideality factor and series resistance values. Low leakage currents in the order of ~30 nA at −1 V are consistently measured. Rectification ratios of up to ~10 5 (at ±1 V bias) are achieved. A fitting curve in the diffusion current region reveals ideality factors of n ~1.58. These values can be attributed to several factors. First, the SAE approach does not require any catalyst [34] (for example, gold or copper) to initiate the growth, avoiding any metal incorporation within the GaAs crystal that has been reported to increase the reverse bias leakage current in nanowire-based devices [45] . Second, the high-bandgap InGaP shell minimizes the surface state density on the nanofacets that could partly deplete the inner n–p core–shell junction. This is witnessed by the fact that the ideality factor is far below the space-charge-limited condition ( n ≥2). In high-injection regime, a series resistance R s ~530 Ω is extrapolated from the fitting curve R s = V/I . The NP-based solar cells are then tested under air mass 1.5 global (AM 1.5 G) illumination conditions (calibrated 1,000 W m −2 , 1 sun), at room temperature. Figure 4b illustrates current density versus voltage ( J–V ) characteristics under light for devices with and without in situ epitaxial passivation. For PV devices without InGaP shells (dashed line), open-circuit voltages ( V oc ) of 0.37 V and short-circuit current densities ( J sc ) of 12.8 mA cm −2 with fill factor (FF) of 21% are observed. This translates into PCE of up to 1.02%. The ‘S-shape’ kink in the J–V characteristic is indicative of interfacial effects such as surface dipoles, defects and traps that create barriers for carrier extraction [46] . This effect leads to a loss in both J sc and FF, evidently reducing the PCE of the final device. In case of core–shell junctions capped with InGaP shells, the optoelectronic properties are markedly improved: V oc =0.44 V, J sc =24.3 mA cm −2 and FF=62%. This results into a final PCE of 6.63%. InGaP is reducing surface states as confirmed by high FF and J sc . The V oc value is increased by ~20% compared with un-passivated devices and it is the highest measured in GaAs NP-array PVs. Figure 4: Dark and light characterization of photovoltaic devices. ( a ) Semi-log dark current–voltage characteristic of a typical GaAs NP array. Both ideality factors ( n =1.58, red dots) and high-injection series resistance ( R s ~530 Ω, green dots) are extrapolated by means of fitting curves. The type of carrier transport is well below the space-charge-limited model ( n 2). The good diodic behaviour is corroborated by a 10 4.7 rectification ratio. ( b ) Current density–voltage characteristics under air mass 1.5 global illumination conditions for photovoltaic devices with (solid red line) and without in situ InGaP shell (dashed green line). InGaP-passivated photovoltaic cells show an open-circuit voltage of 0.44 V, short-circuit current density of 24.3 mA cm −2 and FFs of 62%. This translates into a PCE that amounts to 6.63%. Full size image V oc values of ~0.9 V are expected for planar GaAs solar cells [47] . This discrepancy can be attributed to the fact that the surface-state density is being effectively alleviated but not suppressed altogether. From measurements on single GaAs NP-field effect transistors, the surface state densities before and after InGaP surface passivation decreases from 5 × 10 12 cm −2 eV −1 to 7 × 10 10 cm −2 eV −1 , respectively [48] . Furthermore, the measured V oc is a collective figure of merit resulting from ~2.8 × 10 8 p–n junctions per cm 2 (considering a square-lattice arrangement, 600 nm pitch) connected in parallel. For this reason, dopant incorporation inhomogeneities and/or defective NPs within the whole array can severely lower the final V oc at the terminals. The NPs constituting the whole array are required to be almost electrically and optically identical. Recent studies on dopant mapping in NPs, showed doping variations in excess of two orders of magnitude along both axial and radial directions [49] , [50] , [51] , raising clear differences with respect to a canonical abrupt, metallurgical planar p–n junction. 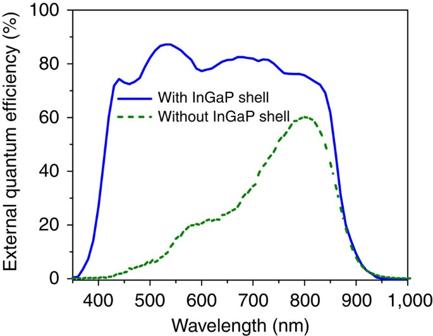Figure 5: Quantum yield comparison. EQE measurements of processed GaAs NP solar cell devices with (solid blue line) and without (dashed green line) wide-bandgapin situpassivation. Figure 5 shows a comparison of external quantum efficiency (EQE) curves for devices with and without passivation. The measurements are taken from 340–1,000 nm. The EQE values for the NP arrays capped with InGaP shells are well above 70% in the spectral regime of interest (blue solid line), with a peak efficiency of ~86% at 520 nm. For bare-grown radial p–n junctions, high-energy photons are possibly recombining at the surface (green dashed line). This is due to the fact that high-energy photons have shorter penetration depths into GaAs compared to infrared photons, therefore being the most sensitive to recombination centres at the surface [52] . Consequently, the EQE response is considerably reduced especially in the ultraviolet-visible spectral region when in situ passivation is not adopted. Table 1 summarizes the most recent results on arras of GaAs NPs employed in PV devices [5] , [6] , [53] . Particular emphasis is dedicated to different contact schemes and passivation techniques employed. To notice it is the dramatic PCE improvement once a high-bandgap passivation technique is introduced. Also, a tested ohmic contact at the transparent electrode/semiconductor interface leads to considerably higher FF values. Figure 5: Quantum yield comparison. EQE measurements of processed GaAs NP solar cell devices with (solid blue line) and without (dashed green line) wide-bandgap in situ passivation. Full size image Table 1 Comparative performance of GaAs nanowire-array photovoltaics. Full size table In conclusion, this work reports the highest efficiency to date for GaAs-based NP-array solar cells employing InGaP in situ passivation with an overall PCE of 6.63% under AM 1.5 G conditions. Thermally annealed Ti/ITO ohmic contacts ensure a good carrier extraction at the top anode while preserving an overall transparency/optical coupling with the NP arrays. Photo-electrical measurements highlight the necessity of an in situ passivation treatment to dramatically improve EQE (above 70%) as well as the total PCE. The array architecture offers a path for a practical large area scaled-up solar cell, in opposition with the pervasive characterization of single-NP PVs. These results lay the ground to considerably higher efficiencies in III–V NP-based photovoltaics and open up a route for NP-based multi-junction architectures by means of a careful investigation of contact interface, surface state density and epitaxial growth of dissimilar materials. GaAs nanowire growth The nanowire growth was carried out in a metal organic chemical vapour deposition reactor (Emcore vertical-flow) using hydrogen carrier gas at 60 torr. The n-doped GaAs NPs were grown at 735 °C. Subsequently, the p-doped shells were grown at 600 °C. Lastly, InGaP shells were also grown at 600 °C. An estimated GaAs core diameter of 180 nm, GaAs shell thickness of 40 nm and InGaP-passivating shell of 5 nm were grown radially, with a final NP height of 1.3 μm. The primary precursors used during growth were tri-methyl-gallium, tertiary-butyl-arsine, trimethyl-indium and tertiary-butyl-phosphorus. The doping sources were tetra-ethyl-tin and di-methyl-zinc as the n-type and p-type dopants, respectively. The tri-methyl-gallium was pressurized to 900 Torr, chilled to 0 °C and had a hydrogen flow rate of 3 s.c.c.m. The tertiary-butyl-arsine was pressurized to 700 Torr, chilled to 20 °C and with a hydrogen flow rate of 10 s.c.c.m. Device fabrication Subsequent to growth, the GaAs nanowire arrays were cleaned in acetone, methanol and isopropanol for 1 min each. Native oxide was removed by using an aqueous ammonium hydroxide (NH 4 OH:H 2 O, 1:30) solution for 30 s. Ohmic gold-germanium/nickel/gold (200 nm/40 nm/100 nm) back metal contacts were electron-beam evaporated on the dies and thermally annealed at 400 °C for 30 s. BCB (Cyclotene Dow Chemical) was spin coated as purchased at 3,000 r.p.m. for 30 s and hard cured overnight at 250 °C. BCB was then etched back using CF 4 /O 2 reactive ion plasma etch chemistry (Oxford 80 Plus) at a rate of 3.5 nm s −1 . InGaP at the NP tips was chemically removed by a selective wet etch (H 3 PO 4 :HCl, 7:1). Titanium (from Kurt J. Lesker) was deposited as a transparent interlayer between the semiconductor interface and the subsequent layer in DC magnetron sputtering mode at 75 W (Ulvac JSP 8000) at a low rate of 1 nm min −1 to achieve a continuous metallic thin film at room temperature, 30 s.c.c.m. of argon gas. Indium tin oxide (from Kurt J. Lesker) was deposited as transparent layer right after the Ti interlayer during the same run in RF magneton-sputtering mode (Ulvac JSP 8000) at 300 W at a rate of 8 nm min −1 at room temperature and 10 s.c.c.m. of argon gas, 0.5 s.c.c.m. of oxigen gas. All the depositions were carried out at 0.65 mT pressure. Rapid thermal annealing (RTP-600xp) was performed at 300 °C for 1 min in an Argon-purged atmosphere. For optical transmittance, the transparent films were deposited on quartz slides and measured by means of Fourier transform infrared spectroscopy (UV–vis-NIR ISR-3100). Solar cell characterization Current–voltage characteristics of the transparent contacts and solar cells were measured using a source metre (Keithley 2400). AM 1.5 illumination was carried out with a 300-W xenon-lamp-based solar simulator (Newport Corporation, 67005) with an AM 1.5 G filter mounted. The light intensity was calibrated using a 1-sun (1,000 W m −2 ) reference silicon photodiode. The EQE spectra were acquired by using a manufactured EQE set-up (Newport Corporation, 74125) equipped with a 1-sun bias, monochromator, lock-in amplifier for the photocurrent acquisition and calibrated silicon photodiode (Newport Corporation, 70356). Power density and spectral mismatch were further monitored using a calibrated reference solar cell. The estimated error in the EQE measurement amounts to ±1.5%. The monochromatic illumination step was 5 nm. An objective lens with a focal length of 100 mm was used to focus down the spot size. How to cite this article: Mariani G. et al . GaAs nanopillar-array solar cells employing in situ surface passivation. Nat. Commun. 4:1497 doi: 10.1038/ncomms2509 (2013).